The neuritic plaque facilitates pathological conversion of tau in an Alzheimer’s disease mouse model A central question in Alzheimer’s Disease (AD) is whether the neuritic plaque is necessary and sufficient for the development of tau pathology. Hyperphosphorylation of tau is found within dystrophic neurites surrounding β-amyloid deposits in AD mouse models but the pathological conversion of tau is absent. Likewise, expression of a human tau repeat domain in mice is insufficient to drive the pathological conversion of tau. Here we developed an Aβ-amyloidosis mouse model that expresses the human tau repeat domain and show that in these mice, the neuritic plaque facilitates the pathological conversion of wild-type tau. We show that this tau fragment seeds the neuritic plaque-dependent pathological conversion of wild-type tau that spreads from the cortex and hippocampus to the brain stem. These results establish that in addition to the neuritic plaque, a second determinant is required to drive the conversion of wild-type tau. Alzheimer’s disease (AD), the most common cause of dementia, is pathologically characterized by the accumulation of neuritic plaques and neurofibrillary tangles (NFT), with widespread gliosis, loss of synapses and degeneration of neurons [1] , [2] . The core of neuritic plaques consists of extracellular deposits of Aβ [3] surrounded by astrocytes and microglia. The NFT is comprised of intracellular paired helical filaments derived from hyperphosphorylated microtubule binding protein, tau [4] , [5] . Genetic studies of early-onset familial AD (fAD), which accounts for 5–10% of cases of AD [6] , [7] , have fuelled the notion that abnormal accumulation of Aβ in the brain would trigger the aggregation of tau leading to neurodegeneration and dementia [2] , [8] . While previous studies showed that accumulation of Aβ could facilitate tau aggregation in FTDP-17 linked mutant Tau mice [9] , [10] , [11] , [12] , [13] , no such evidence have been demonstrated using a non-mutant tau model. Furthermore, it is not known whether the neuritic plaque is necessary and sufficient to drive the conversion of wild-type tau. In contrast to mutations in APP and Presenilins linked to fAD [14] , [15] , genetic risk alleles, including ApoE [16] , [17] , [18] , [19] and Trem2 (refs 20 , 21 ), are associated with late-onset AD (LOAD), which constitutes ∼ 90% of AD cases. The notion that accumulation of Aβ is not sufficient to drive cognitive decline in LOAD is strongly supported by the following: a high Aβ burden is found in brains of some elderly in their eighties or nineties who remain cognitively normal [22] , [23] , [24] ; and there is no correlation of Aβ plaques with cognition in LOAD [25] . In contrast, the aggregation of tau correlates with cognitive decline and is thought to drive neurodegeneration in AD [26] , [27] . This raises the intriguing notion that in addition to the Aβ burden, other risk factors help provoke the pathological conversion of tau to drive neuron loss and cognitive decline in LOAD. Resolution of this question will impact our view regarding disease mechanisms and identification of targets, and validate and test novel therapeutic strategies for LOAD. Animal model systems have been instrumental in clarifying the molecular mechanisms and testing therapeutic strategies for AD [28] , [29] , [30] , [31] , [32] , [33] . Notwithstanding advances made using current rodent models [10] , [34] , [35] , [36] , [37] , [38] , [39] , [40] , a major limitation in the field is the lack of a rodent model that faithfully reproduce the tau pathology seen in humans with AD. Because no mutation in the tau gene has been identified in fAD or LOAD patients and expression of human wild-type tau failed to elicit tau pathology [41] , current mouse models of tau pathology are primarily based on transgenes expressing tau mutants linked to FTDP-17 (refs 9 , 10 , 11 , 35 , 36 , 37 , 42 ). However, this raises major concerns regarding their relevance to the disease context. It is well recognized that the tau pathology occurring in AD invariably depends on the conversion of the wild-type tau, a prion strain that is distinct from other human tauopathies such as that associated with FTDP-17 (ref. 43 ). Moreover, the tau pathology occurring in these FTDP-17-linked tau models is sufficient to drive cell death independent of Aβ plaques [44] , supporting the view that these mice may be good models of FTDP-17, but not of AD. To address this critical unmet need, we developed a mouse model in which wild-type tau is converted into pathological tau aggregates and NFT that are propagated through neuronal circuits to drive neuron loss in a neuritic plaque-dependent manner. Our results offer novel mechanistic insight for the pathogenesis of AD. Neuritic plaque is not sufficient for the conversion of tau Although it is well recognized that endogenous tau can be hyperphosphorylated in mouse models of β-amyloidosis [40] , whether the neuritic plaque is necessary and sufficient to facilitate the pathological conversion of wild-type tau is not known. To address this issue, we examined first the biochemical alterations of endogenous tau occurring in APP swe ;PS1ΔE9 mice (a well-established mouse model of β-amyloidosis) during aging. Correlated with the presence of neuritic plaques was hyperphosphorylation of tau occurring within dystrophic neurites ( Fig. 1a ). The hyperphosphorylated tau was seen surrounding the central Aβ core but never co-localized with it ( Fig. 1b ); while closely associated, there is no direct physical interaction between the central Aβ core and the hyperphosphorylated tau. Moreover, the hyperphosphorylated tau was localized adjacent to ubiquitinated proteins within dystrophic neurites ( Fig. 1c ). Because tau was not hyperphosphorylated before the formation of neuritic plaques and its biochemical alteration persisted during aging ( Fig. 1d,e ), we infer that the neuritic plaque serves as the crucible that facilitates the hyperphosphorylation of tau. However, this persistent neuritic plaque-dependent biochemical alteration of tau failed to convert to tangle-like aggregates even in aged APP swe ;PS1ΔE9 mice that were beyond 24 months as judged by Gallyas preparation ( Fig. 1f ), a silver stain method for detecting conformational changes in tau. While the neuritic plaque is capable of stimulating the phosphorylation of tau, it is not sufficient to alter the conformation of tau to form tangles and drive the loss of neurons. 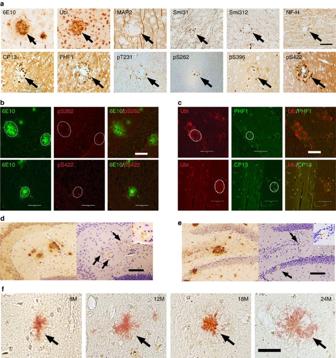Figure 1: Neuritic plaques stimulate the phosphorylation of tau. (a) Brain sections ofAPPswe;PS1ΔE9mice (n=7) were detected by antibodies specific to Aβ (6E10), ubiquitin, Microtubule-associated protein 2 (Map2), neurofilament (Smi31, Smi312, and NF-H), and antibodies specific to phosphorylated tau: CP13 and PHF-1, Tau pT231, Tau pS262, Tau pS396, and Tau-pS422. Note the accumulation of phosphorylated tau surrounding the neuritic plaques. Scale bar, 50 μm. (b) Confocal microscopic analysis of Aβ and tau in cortex ofAPPswe;PS1ΔE9mice (n=6). Brain sections co-stained with antiserums specific to: Aβ (6E10) and tau (pS262) (upper panel); or Aβ (6E10) and tau (pS422) (lower panel). Scale bar, 50 μm. (c) Confocal microscopic analysis of Ubiquitin and tau in cortex ofAPP;PS1ΔE9mice (n=6). Brain sections co-stained with antiserums specific to: Ubiquitin and tau (CP13) (upper panel); or Ubiquitin and PHF-1 (lower panel). Scale bar, 50 μm. (d) Accumulation of phosphorylated tau in dystrophic neurites surrounding the central Aβ core in 6-month-oldAPPswe;PS1ΔE9mice (n=9) as detected by antibodies specific to Aβ (6E10) and phosphorylated tau (pS422). Scale bar, 100 μm. (e) Accumulation of phosphorylated tau in dystrophic neurites surrounding the central Aβ core in 12-month-oldAPPswe;PS1ΔE9mice (n=11) as detected by antibodies specific to Aβ (6E10) and phosphorylated tau (pS422). Scale bar, 100 μm. (f) No Gallyas positive tau tangle was detected around the Aβ core of neuritic plaques (Congo red, arrows) inAPPswe;PS1ΔE9mice (n=9), even up to 24 months. Scale bar, 25 μm. Figure 1: Neuritic plaques stimulate the phosphorylation of tau. ( a ) Brain sections of APP swe ;PS1ΔE9 mice ( n =7) were detected by antibodies specific to Aβ (6E10), ubiquitin, Microtubule-associated protein 2 (Map2), neurofilament (Smi31, Smi312, and NF-H), and antibodies specific to phosphorylated tau: CP13 and PHF-1, Tau pT231, Tau pS262, Tau pS396, and Tau-pS422. Note the accumulation of phosphorylated tau surrounding the neuritic plaques. Scale bar, 50 μm. ( b ) Confocal microscopic analysis of Aβ and tau in cortex of APP swe ;PS1ΔE9 mice ( n =6). Brain sections co-stained with antiserums specific to: Aβ (6E10) and tau (pS262) (upper panel); or Aβ (6E10) and tau (pS422) (lower panel). Scale bar, 50 μm. ( c ) Confocal microscopic analysis of Ubiquitin and tau in cortex of APP;PS1ΔE9 mice ( n =6). Brain sections co-stained with antiserums specific to: Ubiquitin and tau (CP13) (upper panel); or Ubiquitin and PHF-1 (lower panel). Scale bar, 50 μm. ( d ) Accumulation of phosphorylated tau in dystrophic neurites surrounding the central Aβ core in 6-month-old APP swe ;PS1ΔE9 mice ( n =9) as detected by antibodies specific to Aβ (6E10) and phosphorylated tau (pS422). Scale bar, 100 μm. ( e ) Accumulation of phosphorylated tau in dystrophic neurites surrounding the central Aβ core in 12-month-old APP swe ;PS1ΔE9 mice ( n =11) as detected by antibodies specific to Aβ (6E10) and phosphorylated tau (pS422). Scale bar, 100 μm. ( f ) No Gallyas positive tau tangle was detected around the Aβ core of neuritic plaques (Congo red, arrows) in APP swe ;PS1ΔE9 mice ( n =9), even up to 24 months. Scale bar, 25 μm. Full size image Tau repeat domain is insufficient for the conversion of tau The insufficiency of the neuritic plaque to drive the pathological conversion of tau suggested that a second-risk determinant may be required. That accumulating evidence indicated that other types of tau modification, such as fragmentation [45] or acetylation [46] , [47] , facilitate its aggregation encouraged us to determine whether a tau repeat domain could facilitate the pathological conversion of wild-type tau. We used the moPrP-tet vector [48] to express a human four-repeat domain of tau (Q244-E372, TauRD) in the nervous system of mice under the control of the tetracycline transactivator (tTA) ( Fig. 2a ). From multiple lines, we selected for subsequent studies one Tau4R line, which accumulated the human tau fragment to ∼ 1.1-fold of endogenous tau ( Fig. 2b , Supplementary Fig. 1 ). No difference can be detected in the overall structure and weight of brains of Tau4R mice even at 25 months of age ( Fig. 2c , third column). Histological analysis confirmed no evidence of activation of astrocytes/microglia or neuronal loss in Tau4R mice ( Fig. 2d , third column). We also failed to observe hyperphosphorylation of tau or formation of tau tangle ( Fig. 3a,b , forth column), indicating that the tau repeat domain alone is insufficient to drive the pathological conversion of wild-type tau. 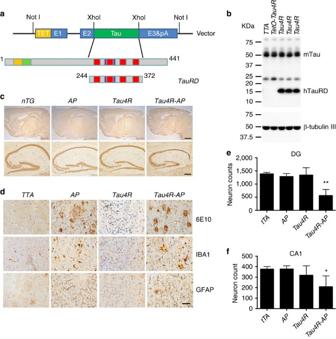Figure 2: Neuritic plaque is required for the pathological conversion of tau. (a) Diagram depicting the expression construct of four-repeat domain of tau (TauRD). The top diagram represents the longest isoform of the human tau40 (441 residues). The bottom diagram shows the construct containing four-repeat domain of tau with (TauRD). (b) Protein blot using 77G7 antibody that recognized the repeat domain of tau showed the presence of exogenous (∼16 kDa) TauRD and endogenous tau protein from brain lysates of tau transgenic (Tau4R) mice (n=5). The expression level of tau inTau4Rmice is similar to that of non-transgenic mice. (c) Immunohistochemical analysis of brains of 20-month-oldnTG(n=5), TTA(n=4), Tau4R(n=6) andTau4R-APmice (n=5) using antiserum specific to NeuN to detect neurons; sagittal sections of brains (upper panels; scale bar, 1,000 μm) and hippocampi (lower panels; scale bar, 200 μm). Note forebrain atrophy and reduction of neurons in the cortical and hippocampal area ofTau4R-APmice. (d) Immunohistochemical analysis using antiserum specific to Aβ (6E10), microglia (IBA1) and reactive astrocytes (GFAP). Scale bar, 50 μm. Immunohistochemial analysis of brains ofnTG(n=5), TTA(n=4), Tau4R(n=6) andTau4R-APmice (n=5) using antiserum specific to Aβ (6E10), microglial (IBA1) and reactive astrocytes (GFAP). Note increase of microglial and hypertrophic GFAP positive astrocytes in cortex of 20-month-oldTau4R-APmice. Scale bar, 50 μm. (e) Neuronal cell count of dentate gyrus region from 18 months oldTTA(n=5),AP(n=5),Tau4R(n=5), Tau4R-AP(n=5) mice using ImageJ analysis. (one-way analysis of variance (ANOVA), **P=0.0002) (f) Neuronal cell count of CA1 regions from 20 months oldTTA(n=4),AP(n=6),Tau4R(n=6), Tau4R-AP(n=5) mice using ImageJ analysis. (one-way ANOVA, *P=0.0134). Figure 2: Neuritic plaque is required for the pathological conversion of tau. ( a ) Diagram depicting the expression construct of four-repeat domain of tau ( TauRD ). The top diagram represents the longest isoform of the human tau40 (441 residues). The bottom diagram shows the construct containing four-repeat domain of tau with ( TauRD ). ( b ) Protein blot using 77G7 antibody that recognized the repeat domain of tau showed the presence of exogenous ( ∼ 16 kDa) TauRD and endogenous tau protein from brain lysates of tau transgenic ( Tau4R ) mice ( n =5). The expression level of tau in Tau4R mice is similar to that of non-transgenic mice. ( c ) Immunohistochemical analysis of brains of 20-month-old nTG ( n =5) , TTA ( n =4) , Tau4R ( n =6) and Tau4R-AP mice ( n =5) using antiserum specific to NeuN to detect neurons; sagittal sections of brains (upper panels; scale bar, 1,000 μm) and hippocampi (lower panels; scale bar, 200 μm). Note forebrain atrophy and reduction of neurons in the cortical and hippocampal area of Tau4R-AP mice. ( d ) Immunohistochemical analysis using antiserum specific to Aβ (6E10), microglia (IBA1) and reactive astrocytes (GFAP). Scale bar, 50 μm. Immunohistochemial analysis of brains of nTG ( n =5) , TTA ( n =4) , Tau4R ( n =6) and Tau4R-AP mice ( n =5) using antiserum specific to Aβ (6E10), microglial (IBA1) and reactive astrocytes (GFAP). Note increase of microglial and hypertrophic GFAP positive astrocytes in cortex of 20-month-old Tau4R-AP mice. Scale bar, 50 μm. ( e ) Neuronal cell count of dentate gyrus region from 18 months old TTA ( n =5), AP ( n =5), Tau4R ( n =5) , Tau4R-AP ( n =5) mice using ImageJ analysis. (one-way analysis of variance (ANOVA), ** P =0.0002) ( f ) Neuronal cell count of CA1 regions from 20 months old TTA ( n =4), AP ( n =6), Tau4R ( n =6) , Tau4R-AP ( n =5) mice using ImageJ analysis. (one-way ANOVA, * P =0.0134). 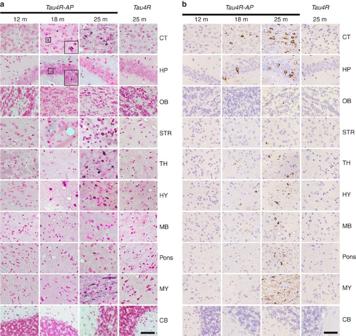Figure 3: Age-dependent spreading of endogenous tau aggregates in brain regions ofTau4R-APmice. (a) Gallyas-Braak silver staining of tau tangles in brain sections ofTau4R-APmice at 12 (n=3), 18 (n=4), and 25 months of age (n=6). The sections were counterstained with fast red. The right panels areTau4Rmice at 25 months of age (n=6). The brain regions are cerebral cortex (CT); hippocampus (HP); olfactory bulb (OB); striatum (STR); thalamus (TH); hypothalamus (HY); midbrain (MB); Pons; Medulla (MY), and cerebellum (CB). Tau tangles could be detected inTau4R-AP, but notTau4R, mice at 18 months of ages, and the accumulation of tangles were dramatically increased with aging and spread to other brain regions (25 months of age, third column), except in cerebellum (bottom panel). Scale bar, 50 μm. (b) Immunohistochemical analysis showed age-dependent spreading of endogenous tau tangle inTau4R-APmice (n=13) using antibodies specific to endogenous phosphorylated S422 of tau (pS422). The brain regions are cerebral cortex (CT); hippocampus (HP); olfactory bulb (OB); striatum (STR); thalamus (TH); hypothalamus (HY); midbrain (MB); Pons; Medulla (MY), and cerebellum (CB). While no signal was detected inTau4Rmice (n=6) even at 25 months of age, tau tangles first appeared in cortical and hippocampal region (18 months of age, second column) ofTau4R-APmice and spread to other brain region with aging (25 months of age, third column), except in cerebellum (bottom panel). Scale bar, 50 μm. Full size image Figure 3: Age-dependent spreading of endogenous tau aggregates in brain regions of Tau4R-AP mice. ( a ) Gallyas-Braak silver staining of tau tangles in brain sections of Tau4R-AP mice at 12 ( n =3), 18 ( n =4), and 25 months of age ( n =6). The sections were counterstained with fast red. The right panels are Tau4R mice at 25 months of age ( n =6). The brain regions are cerebral cortex (CT); hippocampus (HP); olfactory bulb (OB); striatum (STR); thalamus (TH); hypothalamus (HY); midbrain (MB); Pons; Medulla (MY), and cerebellum (CB). Tau tangles could be detected in Tau4R-AP , but not Tau4R , mice at 18 months of ages, and the accumulation of tangles were dramatically increased with aging and spread to other brain regions (25 months of age, third column), except in cerebellum (bottom panel). Scale bar, 50 μm. ( b ) Immunohistochemical analysis showed age-dependent spreading of endogenous tau tangle in Tau4R-AP mice ( n =13) using antibodies specific to endogenous phosphorylated S422 of tau (pS422). The brain regions are cerebral cortex (CT); hippocampus (HP); olfactory bulb (OB); striatum (STR); thalamus (TH); hypothalamus (HY); midbrain (MB); Pons; Medulla (MY), and cerebellum (CB). While no signal was detected in Tau4R mice ( n =6) even at 25 months of age, tau tangles first appeared in cortical and hippocampal region (18 months of age, second column) of Tau4R-AP mice and spread to other brain region with aging (25 months of age, third column), except in cerebellum (bottom panel). Scale bar, 50 μm. Full size image Tau fragment seeds neuritic plaque-dependent tau conversion Although the human tau repeat domain was not sufficient to alter the conformation of endogenous tau, we asked whether such fragmentation of tau could serve as the second-risk determinant in the presence of neuritic plaques to drive tau pathology. To address this question, we crossbred Tau4R mice with APP swe ;PS1ΔE9 mice [49] to generate compound Tau4R;APP swe ;PS1ΔE9 ( Tau4R-AP ) mice. Tau4R-AP mice exhibited marked forebrain atrophy ( Fig. 2c ) with significant neuronal loss in dentate gyrus or CA1 region of the hippocampus, respectively, at 18 ( Fig. 2e ) or 20 ( Fig. 2f ) month of age; the loss of neurons in the cortex and hippocampus is associated with the accumulation of phosphorylated tau and NFT ( Fig. 3a,b ). Taken together with our finding that the neuritic plaque is required for the phosphorylation of tau, these results indicate that the fragmentation of tau could seed the neuritic plaque-dependent pathological conversion of wild-type tau. To access the evolution of tau tangles in Tau4R-AP mice, we performed a time series focusing on the pattern of distribution of mouse tau aggregates. Whereas tau aggregates were undetectable before 1 year of age, they were first detected in hippocampus and cortical regions by 15 months of age and significantly increased by 18 months of age ( Fig. 3a ). By 2 years, tau tangles were readily observed throughout the whole brain except the cerebellum ( Fig. 3a ), suggesting that the tau tangle initiated from the frontal area is able to spread to the rest of the brain through neuronal circuits. Because the pattern and intensity of Gallyas stain paralleled ( Fig. 3a ) those of the immunocytochemical staining of misfolded mouse tau ( Fig. 3b ), these tau tangles would be principally derived from the endogenous tau, especially in the brain stem and midbrain where the human tau fragment was not expressed. These findings indicate that while neither the neuritic plaque nor the human tau repeat domain is sufficient to drive the pathological conversion of wild-type tau, they both are required for the seeding and aggregation of the tau repeat domain, which facilitate the pathological conversion of mouse wild-type tau that spread from the cortex and hippocampus to the brain stem. Neuritic plaque is necessary for the conversion of tau To test directly whether the neuritic plaque is required for the pathological conversion of wild-type tau, we took advantage of the gender difference in onset of neuritic plaques occurring in APP swe ;PS1ΔE9 mice; onset for females or males was, respectively, at 4 or 6 months of age ( Fig. 4 ). We would anticipate that if formation of the neuritic plaque precedes tau pathology, the pathological conversion of wild-type tau should be accelerated; otherwise, no such effect would be expected. For such a test, a mouse model in which the onset of tau pathology occurred after the onset of neuritic plaque in female APP swe ;PS1ΔE9 mice, but similar to that of males, would be necessary. We therefore generated mice expressing the four-repeat domain of tau (Q244-E372) harbouring a pro-aggregation ΔK280 mutation ( Tau4RΔK ), previously shown to induce tau pathology in mice [50] . From multiple lines, we selected one line of Tau4RΔK , in which the exogenous tau fragments accumulated to 0.7-fold of endogenous tau ( Fig. 5a , Supplementary Fig. 1 ). Brains of Tau4RΔK mice showed a progressive and marked atrophy of their forebrains ( Fig. 5b ) accompanied over time by a decline in the weight of brains ( Fig. 5c ). Histopathological analysis confirmed a marked decrease in size of the hippocampus ( Fig. 5d,e ) and cortex ( Fig. 5e ) and a marked reduction in the number of neurons by 12 months of age ( Fig. 5f ). Tau tangles first appeared at 6 months of age ( Fig. 5g , upper panel), which were dramatically increased by 12 months ( Fig. 5g ) and except for the cerebellum, spread throughout the brain ( Fig. 5g , lower panel) by 18 months. Moreover, aggregations derived from the endogenous wild-type tau exhibited a similar pattern ( Fig. 5i ), including the midbrain and brain stem. However, the presence of the human tau fragment was restricted to frontal area of the brain ( Fig. 5h , Supplementary Fig. 2 ), suggesting that the exogenous tau fragment serves as a seed to convert the wild-type tau to tangles, which spread in a prion mechanism to other regions of the brain. 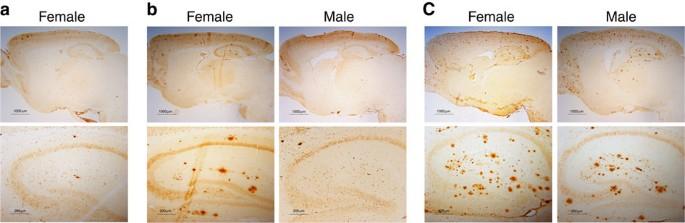Figure 4: Gender difference in onset of neuritic plaques inAPPswe;PS1ΔE9mice. (a) Brain sections of 4-month-old female (n=5)APPswe;PS1ΔE9mice were detected by antibodies specific to Aβ (6E10). Only a few can be detected in the femaleAPPswe;PS1ΔE9mice at 4 months of age. (b) Brain sections of 6-month-old female (n=6) and male (n=4)APPswe;PS1ΔE9mice were detected by antibodies specific to Aβ (6E10). Wide spread neuritic plaques are observed in femaleAPPswe;PS1ΔE9mice, while only a few can be detected in the maleAPPswe;PS1ΔE9mice at 6 months of age. (c) Brain sections of 12-month-old female (n=9) and male (n=7)APPswe;PS1ΔE9mice were detected by antibodies specific to Aβ (6E10). Wide spread neuritic plaques are observed in both male and femaleAPPswe;PS1ΔE9mice at this age. Figure 4: Gender difference in onset of neuritic plaques in APP swe ;PS1ΔE9 mice. ( a ) Brain sections of 4-month-old female ( n =5) APP swe ;PS1ΔE9 mice were detected by antibodies specific to Aβ (6E10). Only a few can be detected in the female APP swe ;PS1ΔE9 mice at 4 months of age. ( b ) Brain sections of 6-month-old female ( n =6) and male ( n =4) APP swe ;PS1ΔE9 mice were detected by antibodies specific to Aβ (6E10). Wide spread neuritic plaques are observed in female APP swe ;PS1ΔE9 mice, while only a few can be detected in the male APP swe ;PS1ΔE9 mice at 6 months of age. ( c ) Brain sections of 12-month-old female ( n =9) and male ( n =7) APP swe ;PS1ΔE9 mice were detected by antibodies specific to Aβ (6E10). Wide spread neuritic plaques are observed in both male and female APP swe ;PS1ΔE9 mice at this age. 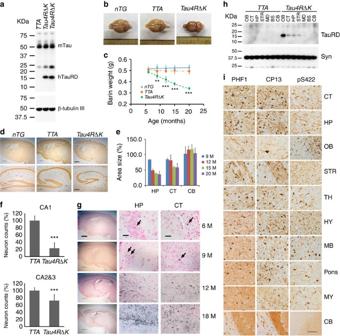Figure 5: Pathological conversion of tau induced by a mutant tau repeat domain. (a) Protein blot using 77G7 antibody to detect exogenous (∼16 kDa) TauRDΔK and endogenous tau protein from brain lysates of mutant tau transgenic (Tau4RΔK) mice (n=9). (b) Representative brains ofnTG, TTA and Tau4RΔKmice at 20 months of age. Note marked forebrain atrophy inTau4RΔKmice (n=7). (c) The plot of brain weight ofnTG(n=29), TTA(n=27) andTau4RΔK(n=24) mice at different of ages. The brain weight ofTau4RΔKmice is progressively reduced with aging. (one-way analysis of variance (ANOVA), 9 M **P=0.02; 12 M ***P=0.0001; 15 M ***P=0.0003; 20 M ***P=0.0006). (d) Immunohistochemical analysis using antiserum specific to NeuN: sagittal sections (upper panels; scale bar, 1,000 μm) and hippocampi (lower panels; scale bar, 200 μm) of 18-month-oldTau4RΔK(n=8) and control mice (n=15). (e) Sizes of cortical (CT), hippocampal (HP) and cerebellum (CB) regions in brains ofTau4RΔK(n=24) at various ages. Note reduction of hippocampus and cortical region, but not cerebellum inTau4RΔKmice. (f) Neuronal cell count of CA1 (T-Test, ***P=4.45E−09) and CA2&3 (T-Test, ***P=0.00033) region from 12 months oldTTA(n=7), Tau4RΔK(n=7) mice using ImageJ analysis. (g) Gallyas-Braak silver staining of brain sections ofTau4RΔKmice at various ages. The sections were counterstained with fast red. The left panel is overview image of the sagittal section of brains (Scale bar, 1,000 μm). The middle and right panels are hippocampal (HP) and cortical regions (CT). (Scale bar, 25 μm). Tau tangle could first be detected at 6 months of age, and the accumulation of tangles were dramatically increased while aging. (h) Total protein was extracted from different brain regions: olfactory bulb (OB), cortex (CT), hippocampus (HP), striatum (STR), midbrain (MB), brain stem (BS), cerebellum (CE) of 9 months oldTTA(n=3) andTau4RΔK(n=3) mice. Human tau fragment (∼16 kDa) detected using anti-human tau polyclonal antiserum KJ9A was only seen in frontal region, but not in MB, BS or CE. (i) Immunohistochemial analysis of brains of 20 months oldTau4RΔKmice (n=5) by antibodies specific to phosphorylated endogenous tau: PHF-1 (left panel), CP13 (middle panel), and tau-pS422 (right panel), respectively. Scale bar, 50 μm. Full size image Figure 5: Pathological conversion of tau induced by a mutant tau repeat domain. ( a ) Protein blot using 77G7 antibody to detect exogenous ( ∼ 16 kDa) TauRDΔK and endogenous tau protein from brain lysates of mutant tau transgenic ( Tau4RΔK ) mice ( n =9). ( b ) Representative brains of nTG, TTA and Tau4RΔK mice at 20 months of age. Note marked forebrain atrophy in Tau4RΔK mice ( n =7). ( c ) The plot of brain weight of nTG ( n =29) , TTA ( n =27) and Tau4RΔK ( n =24) mice at different of ages. The brain weight of Tau4RΔK mice is progressively reduced with aging. (one-way analysis of variance (ANOVA), 9 M ** P =0.02; 12 M *** P =0.0001; 15 M *** P =0.0003; 20 M *** P =0.0006). ( d ) Immunohistochemical analysis using antiserum specific to NeuN: sagittal sections (upper panels; scale bar, 1,000 μm) and hippocampi (lower panels; scale bar, 200 μm) of 18-month-old Tau4RΔK ( n =8) and control mice ( n =15). ( e ) Sizes of cortical (CT), hippocampal (HP) and cerebellum (CB) regions in brains of Tau4RΔK ( n =24) at various ages. Note reduction of hippocampus and cortical region, but not cerebellum in Tau4RΔK mice. ( f ) Neuronal cell count of CA1 ( T -Test, *** P =4.45E −09 ) and CA2&3 ( T -Test, *** P =0.00033) region from 12 months old TTA ( n =7) , Tau4RΔK ( n =7) mice using ImageJ analysis. ( g ) Gallyas-Braak silver staining of brain sections of Tau4RΔK mice at various ages. The sections were counterstained with fast red. The left panel is overview image of the sagittal section of brains (Scale bar, 1,000 μm). The middle and right panels are hippocampal (HP) and cortical regions (CT). (Scale bar, 25 μm). Tau tangle could first be detected at 6 months of age, and the accumulation of tangles were dramatically increased while aging. ( h ) Total protein was extracted from different brain regions: olfactory bulb (OB), cortex (CT), hippocampus (HP), striatum (STR), midbrain (MB), brain stem (BS), cerebellum (CE) of 9 months old TTA ( n =3) and Tau4RΔK ( n =3) mice. Human tau fragment ( ∼ 16 kDa) detected using anti-human tau polyclonal antiserum KJ9A was only seen in frontal region, but not in MB, BS or CE. ( i ) Immunohistochemial analysis of brains of 20 months old Tau4RΔK mice ( n =5) by antibodies specific to phosphorylated endogenous tau: PHF-1 (left panel), CP13 (middle panel), and tau-pS422 (right panel), respectively. Scale bar, 50 μm. Full size image Because the onset of tau pathology in Tau4RΔK mice occurs after the onset of neuritic plaque formation in the female APP swe ;PS1ΔE9 mice ( ∼ 4 months of age, Fig. 4a ), but earlier or at the same time as that of males ( ∼ 6 months of age, Fig. 4b ), we took advantage of this sex difference to determine whether neuritic plaques could accelerate the conversion of wild-type tau to tangles. We crossbred Tau4RΔK mice with APP swe ;PS1ΔE9 mice [49] to generate compound Tau4RΔK;APP swe ;PS1ΔE9 ( Tau4RΔK-AP ) mice. The expression level of exogenous tau in Tau4RΔK-AP mice was comparable to that of the Tau4RΔK mice ( Fig. 6a , Supplementary Fig. 3 ), indicating that the Aβ burden did not influence the expression of tau. Compared with female APP swe ;PS1ΔE9 mice, the amount of Aβ deposit in 6-month-old female Tau4RΔK-AP mice remained unchanged ( Fig. 6c ). As expected, we observed marked increase in accumulation of phosphorylated tau in female Tau4RΔK-AP mice by 6 months of age ( Fig. 6d ). By 9 months of age, female Tau4RΔK-AP mice exhibited marked reduction in brain size ( Fig. 6b ) accompanied by widespread Aβ and tau pathologies ( Fig. 6e,f ). Histological analysis confirmed accelerated atrophy of forebrains in 9-month-old female Tau4RΔK-AP mice( Fig. 7a,b ); specifically, sizes of hippocampus and cortex were significantly reduced ( Fig. 7c,d ). As expected, the cerebellum ( Fig. 7e ) of these Tau4RΔK-AP mice remained normal as tau pathology was absent in this region. To determine the impact of neuritic plaques, we examined neuron loss in brains of 9 month-old female Tau4RΔK-AP mice ( Fig. 7f ). As expected, marked reduction in number of neurons was observed in the cortical and hippocampal area of 9-month-old female Tau4RΔK-AP , but not female Tau4RΔK mice ( Fig. 7g,h ). An 80% and 25% reduction, respectively, in number of neurons were observed in CA1 ( Fig. 7g ) as well as CA2 and CA3 regions ( Fig. 7h ). Moreover, the development of phosphorylated tau aggregates ( Fig. 6g ) and tau tangles ( Fig. 6h ) was greatly accelerated in female Tau4RΔK-AP mice. Using Gallyas silver staining, we observed as early as 9 months of age tau tangles that already spread to the brain stem of Tau4RΔK-AP , but not Tau4RΔK , mice ( Fig. 8a,c,d ); tau tangles in Tau4RΔK mice were seen only at a later time point and by 12 months of age, a greater tau burden was found throughout the brain of Tau4RΔK-AP mice ( Fig. 8b,c,e ). Hypertrophic GFAP positive astrocytes were observed in cortical regions of Tau4RΔK-AP , but not Tau4RΔK , mice ( Fig. 7i ), indicating that reactive astrogliosis is correlated with the loss of neurons. These results indicate that neuritic plaques accelerate the onset of tau aggregation. 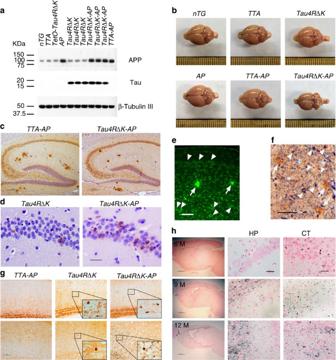Figure 6: Neuritic plaque-dependent acceleration of pathological conversion of tau induced by a mutant tau repeat domain. (a) Protein blot analysis of tau and APP in brain lysates of 3 month-old femaleTTA(n=6), tetO-tauRDΔK(n=6), AP(n=3),TTA-AP(n=7),Tau4RΔK(n=5), Tau4RΔK-AP(n=4) andnTG(n=7) mice using antisera K9JA and CT15. (b) Representative brains of 9 month-old femaleTTA, AP,TTA-AP,Tau4RΔK, Tau4RΔK-APandnTGmice. Note marked forebrain atrophy inTau4RΔKmice. (c) Immunostaining of brain sections of 6-month-old femaleTTA-AP(n=7) andTau4RΔK-APmice (n=5) with antibodies 6E10 specific to human Aβ. Scale bars, 200 μm. (d) Immunostaining of 6 month-old female brain sections ofTau4RΔK(n=4), andTau4RΔK-APmice (n=4) using antiserum tau-pS422. Scale bar, 50 μm. (e) Aβ plaques (arrows) and abundance of tau aggregates (arrowheads) were observed inTau4RΔK-APmice (n=5) at 9 months of age by Thioflavin-T staining. Scale bar, 50 μm. (f) Silver staining to detect Aβ plaques (arrows) and tau tangles (arrowheads) in brain ofTau4RΔK-APmice (n=5). Scale bar, 50 μm. (g) Immunostaining of brain sections of 9 month-old femaleTau4RΔK(n=5), andTau4RΔK-APmice (n=4) using tau-pS422. Scale bar, 100 μm. (h) Gallyas-Braak silver staining of brain sections of femaleTau4RΔK-APmice at 6 (top panel,n=4), 9 (middle panel,n=6) and 12 (bottom panel,n=3) months of age (counterstained with fast red). The left panel: sagittal section (Scale bar, 1,000 μm); middle and right panel are hippocampal (HP) and cortical regions (CT), respectively (Scale bar, 25 μm). Figure 6: Neuritic plaque-dependent acceleration of pathological conversion of tau induced by a mutant tau repeat domain. ( a ) Protein blot analysis of tau and APP in brain lysates of 3 month-old female TTA ( n =6) , tetO-tauRDΔK ( n =6) , AP ( n =3), TTA-AP ( n =7), Tau4RΔK ( n =5) , Tau4RΔK-AP ( n =4) and nTG ( n =7) mice using antisera K9JA and CT15. ( b ) Representative brains of 9 month-old female TTA, AP , TTA-AP , Tau4RΔK, Tau4RΔK-AP and nTG mice. Note marked forebrain atrophy in Tau4RΔK mice. ( c ) Immunostaining of brain sections of 6-month-old female TTA-AP ( n =7) and Tau4RΔK-AP mice ( n =5) with antibodies 6E10 specific to human Aβ. Scale bars, 200 μm. ( d ) Immunostaining of 6 month-old female brain sections of Tau4RΔK ( n =4), and Tau4RΔK-AP mice ( n =4) using antiserum tau-pS422. Scale bar, 50 μm. ( e ) Aβ plaques (arrows) and abundance of tau aggregates (arrowheads) were observed in Tau4RΔK-AP mice ( n =5) at 9 months of age by Thioflavin-T staining. Scale bar, 50 μm. ( f ) Silver staining to detect Aβ plaques (arrows) and tau tangles (arrowheads) in brain of Tau4RΔK-AP mice ( n =5). Scale bar, 50 μm. ( g ) Immunostaining of brain sections of 9 month-old female Tau4RΔK ( n =5), and Tau4RΔK-AP mice ( n =4) using tau-pS422. Scale bar, 100 μm. ( h ) Gallyas-Braak silver staining of brain sections of female Tau4RΔK-AP mice at 6 (top panel, n =4), 9 (middle panel, n =6) and 12 (bottom panel, n =3) months of age (counterstained with fast red). The left panel: sagittal section (Scale bar, 1,000 μm); middle and right panel are hippocampal (HP) and cortical regions (CT), respectively (Scale bar, 25 μm). 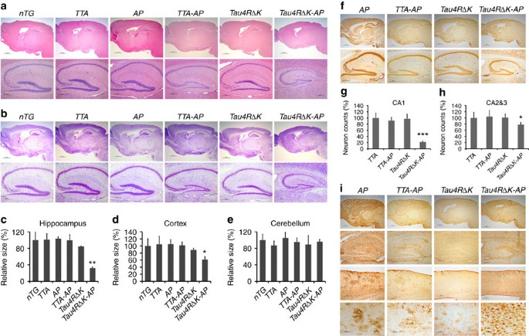Figure 7: Acceleration of neuronal loss, astrocytosis and forebrain atrophy inTau4RΔK-APmice. (a) Hematoxylin and eosin (H&E) staining of sagittal sections of brains (upper panels; scale bar, 1,000 μm) and hippocampi (lower panels; scale bar, 200 μm) of 9-month-old femaleTTA, APPswe;PS1ΔE9(AP),TTA;APPswe;PS1ΔE9(TTA-AP),Tau4RΔK, Tau4RΔK;APPswe;PS1ΔE9(Tau4RΔK-AP) and non-transgenic(nTG)mice. Note forebrain atrophy and reduction of neurons in the cortical and hippocampal area ofTau4RΔK-APmice. (b) Cresyl violet (CV) staining of sagittal sections of brains (upper panels; scale bar, 1,000 μm) and hippocampi (lower panels; scale bar, 200 μm) of 9-month-old femaleTTA, APPswe;PS1ΔE9(AP),TTA;APPswe;PS1ΔE9(TTA-AP),Tau4RΔK, Tau4RΔK;APPswe;PS1ΔE9(Tau4RΔK-AP) and non-transgenic(nTG)mice. Note reduction of neurons inTau4RΔK-APmice. (c–e) Sizes of hippocampal (c), cortical (d) and cerebellum (e) regions in brains of 9 months oldTTA(n=6), AP(n=7),TTA-AP(n=6),Tau4RΔK(n=5), Tau4RΔK-AP(n=4) andnTG(n=15). Note reduction of hippocampus (one-way analysis of variance (ANOVA), **P=0.00052) and cortical region (one-way ANOVA, *P=0.014), but not cerebellum inTau4RΔK-APmice (f) Immunohistochemical analysis of brains of 9 months oldAPPswe;PS1ΔE9,TTA-AP,Tau4RΔKandTau4RΔK-APmice using antiserum specific to NeuN to detect neurons; sagittal sections of brains (upper panels; scale bar, 1,000 μm) and hippocampi (lower panels; scale bar, 200 μm). Note forebrain atrophy and reduction of neurons in the cortical and hippocampal area ofTau4RΔK-APmice. (g) Neuronal cell count of CA1 region from 9 months oldTTA(n=5),TTA-AP(n=6),Tau4RΔK(n=5), Tau4RΔK-AP(n=5) mice using ImageJ analysis. Note∼80% reduction of neurons inTau4RΔK-APmice. (***, One-way ANOVA,P=2.04E-06) (h) Neuronal cell count of CA2 and CA3 regions from 9 months old mice using ImageJ analysis. Significant reduction (∼20%) of neurons are observed ofTau4RΔK-APmice as compared with those of control mice. (one-way ANOVA, *P=0.0133) (i) Immunohistochemial analysis of brains ofAPPswe;PS1ΔE99,TTA-AP, Tau4RΔKandTau4RΔK-APmice at 9 months of age using antiserum against GFAP: sagittal section (top panel, scale bar, 1,000 μm); hippocampi (second panel, scale bar, 200 μm); cortex (third panel, scale bar, 200 μm); higher power views of cortex (fourth panel, scale bar, 50 μm). Note hypertrophic GFAP positive astrocytes in cortex ofTau4RΔK-APmice. Full size image Figure 7: Acceleration of neuronal loss, astrocytosis and forebrain atrophy in Tau4RΔK-AP mice. ( a ) Hematoxylin and eosin (H&E) staining of sagittal sections of brains (upper panels; scale bar, 1,000 μm) and hippocampi (lower panels; scale bar, 200 μm) of 9-month-old female TTA, APP swe ;PS1ΔE9(AP) , TTA;APP swe ;PS1ΔE9 ( TTA-AP ), Tau4RΔK, Tau4RΔK;APP swe ;PS1ΔE9 ( Tau4RΔK-AP ) and non-transgenic (nTG) mice. Note forebrain atrophy and reduction of neurons in the cortical and hippocampal area of Tau4RΔK-AP mice. ( b ) Cresyl violet (CV) staining of sagittal sections of brains (upper panels; scale bar, 1,000 μm) and hippocampi (lower panels; scale bar, 200 μm) of 9-month-old female TTA, APP swe ;PS1ΔE9(AP) , TTA;APP swe ;PS1ΔE9 ( TTA-AP ), Tau4RΔK, Tau4RΔK;APP swe ;PS1ΔE9 ( Tau4RΔK-AP ) and non-transgenic (nTG) mice. Note reduction of neurons in Tau4RΔK-AP mice. ( c – e ) Sizes of hippocampal ( c ), cortical ( d ) and cerebellum ( e ) regions in brains of 9 months old TTA ( n =6) , AP ( n =7), TTA-AP ( n =6), Tau4RΔK ( n =5) , Tau4RΔK-AP ( n =4) and nTG ( n =15). Note reduction of hippocampus (one-way analysis of variance (ANOVA), ** P =0.00052) and cortical region (one-way ANOVA, * P =0.014), but not cerebellum in Tau4RΔK-AP mice ( f ) Immunohistochemical analysis of brains of 9 months old APP swe ;PS1ΔE9 , TTA-AP , Tau4RΔK and Tau4RΔK-AP mice using antiserum specific to NeuN to detect neurons; sagittal sections of brains (upper panels; scale bar, 1,000 μm) and hippocampi (lower panels; scale bar, 200 μm). Note forebrain atrophy and reduction of neurons in the cortical and hippocampal area of Tau4RΔK-AP mice. ( g ) Neuronal cell count of CA1 region from 9 months old TTA ( n =5), TTA-AP ( n =6), Tau4RΔK ( n =5) , Tau4RΔK-AP ( n =5) mice using ImageJ analysis. Note ∼ 80% reduction of neurons in Tau4RΔK-AP mice. (***, One-way ANOVA, P =2.04E-06) ( h ) Neuronal cell count of CA2 and CA3 regions from 9 months old mice using ImageJ analysis. Significant reduction ( ∼ 20%) of neurons are observed of Tau4RΔK-AP mice as compared with those of control mice. (one-way ANOVA, * P =0.0133) ( i ) Immunohistochemial analysis of brains of APP swe ;PS1ΔE99 , TTA-AP, Tau4RΔK and Tau4RΔK-AP mice at 9 months of age using antiserum against GFAP: sagittal section (top panel, scale bar, 1,000 μm); hippocampi (second panel, scale bar, 200 μm); cortex (third panel, scale bar, 200 μm); higher power views of cortex (fourth panel, scale bar, 50 μm). Note hypertrophic GFAP positive astrocytes in cortex of Tau4RΔK-AP mice. 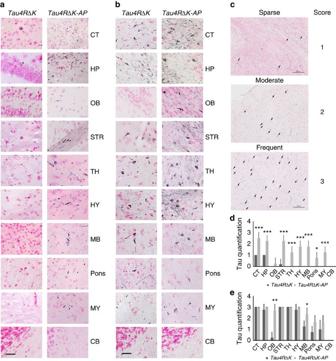Figure 8: Acceleration of tau pathology in femaleTau4RΔK-APmice. (a) Gallyas-Braak silver staining of brain sections of femaleTau4RΔK(n=5) andTau4RΔK-APmice (n=4) at 9 months of age (counterstained with fast red). Cerebral cortex (CT); hippocampus (HP); olfactory bulb (OB); striatum (STR); thalamus (TH); hypothalamus (HY); midbrain (MB); Pons; Medulla (MY), and cerebellum (CB) were shown, respectively. While only sparse tau tangle was detected in frontal area of theTau4RΔKmice, wide spread tau tangle and thread were observed inTau4RΔK-APmice, including brain stem. (Scale bar, 25 μm). (b) Gallyas-Braak silver staining of brain sections of femaleTau4RΔK(n=4) andTau4RΔK-APmice (n=3) at 12 months of age (counterstained with fast red). Cerebral cortex (CT); hippocampus (HP); olfactory bulb (OB); striatum (STR); thalamus (TH); hypothalamus (HY); midbrain (MB); Pons; Medulla (MY), and cerebellum (CB) were shown, respectively. Note more tau tangles were detected in different brain regions ofTau4RΔK-APmice as compare with that ofTau4RΔKmice. (Scale bar, 25 μm). (c) Semiquantificative score of tau tangle frequency in low power (200X) microscope field. Score was indicated as: 0, no tangle; 1, 1–5 tangles per field; 2, 6–15 tangles per field; and 3, >15 tangles per field. (Scale bar, 100 μm) (d) Score of tau tangle frequency in different brain regions of 9 months old femaleTau4RΔK(n=5) andTau4RΔK-AP(n=4) mice. Cerebral cortex (CT;T-Test, ***P=0.0006); hippocampus (HP;T-Test, ***P=0.0007); olfactory bulb (OB); striatum (STR;T-Test, ***P=0.0003); thalamus (TH;T-Test, ***P=0.0007); hypothalamus (HY;T-Test, ***P=0.0001); midbrain (MB;T-Test, ***P=0.0001); Pons(T-Test, *P=0.01); Medulla (MY;T-Test, ***P=0.0007), and cerebellum (CB) were shown. While tau tangles were only detected in frontal region inTau4RΔKmice, widespread tau tangles were observed in whole brain ofTau4RΔK-APmice, including brain stem. (e) Score of tau tangle frequency in different brain regions of 12 months old femaleTau4RΔK(n=4) andTau4RΔK-AP(n=3) mice. CT; HP; OB (T-Test, **P=0.002); STR; TH; HY; MB, (T-Test, *P=0.045); Pons; MY, and CB region were shown. Note more frequent tau tangles detected in different regions ofTau4RΔK-APmice compared with that ofTau4RΔKmice, especially in olfactory bulb and brain stem. Full size image Figure 8: Acceleration of tau pathology in female Tau4RΔK-AP mice. ( a ) Gallyas-Braak silver staining of brain sections of female Tau4RΔK ( n =5) and Tau4RΔK-AP mice ( n =4) at 9 months of age (counterstained with fast red). Cerebral cortex (CT); hippocampus (HP); olfactory bulb (OB); striatum (STR); thalamus (TH); hypothalamus (HY); midbrain (MB); Pons; Medulla (MY), and cerebellum (CB) were shown, respectively. While only sparse tau tangle was detected in frontal area of the Tau4RΔK mice, wide spread tau tangle and thread were observed in Tau4RΔK-AP mice, including brain stem. (Scale bar, 25 μm). ( b ) Gallyas-Braak silver staining of brain sections of female Tau4RΔK ( n =4) and Tau4RΔK-AP mice ( n =3) at 12 months of age (counterstained with fast red). Cerebral cortex (CT); hippocampus (HP); olfactory bulb (OB); striatum (STR); thalamus (TH); hypothalamus (HY); midbrain (MB); Pons; Medulla (MY), and cerebellum (CB) were shown, respectively. Note more tau tangles were detected in different brain regions of Tau4RΔK-AP mice as compare with that of Tau4RΔK mice. (Scale bar, 25 μm). ( c ) Semiquantificative score of tau tangle frequency in low power (200X) microscope field. Score was indicated as: 0, no tangle; 1, 1–5 tangles per field; 2, 6–15 tangles per field; and 3, >15 tangles per field. (Scale bar, 100 μm) ( d ) Score of tau tangle frequency in different brain regions of 9 months old female Tau4RΔK ( n =5) and Tau4RΔK-AP ( n =4) mice. Cerebral cortex (CT; T -Test, *** P =0.0006); hippocampus (HP; T -Test, *** P =0.0007); olfactory bulb (OB); striatum (STR; T -Test, *** P =0.0003); thalamus (TH; T -Test, *** P =0.0007); hypothalamus (HY; T -Test, *** P =0.0001); midbrain (MB; T -Test, *** P =0.0001); Pons( T -Test, * P =0.01); Medulla (MY; T -Test, *** P =0.0007), and cerebellum (CB) were shown. While tau tangles were only detected in frontal region in Tau4RΔK mice, widespread tau tangles were observed in whole brain of Tau4RΔK-AP mice, including brain stem. ( e ) Score of tau tangle frequency in different brain regions of 12 months old female Tau4RΔK ( n =4) and Tau4RΔK-AP ( n =3) mice. CT; HP; OB ( T -Test, ** P =0.002); STR; TH; HY; MB, ( T -Test, * P =0.045); Pons; MY, and CB region were shown. Note more frequent tau tangles detected in different regions of Tau4RΔK-AP mice compared with that of Tau4RΔK mice, especially in olfactory bulb and brain stem. Full size image However, tau pathology was not accelerated in male Tau4RΔK-AP mice as compared with that of Tau4RΔK mice. At 12 months of age, while marked acceleration of brain atrophy was observed in female Tau4RΔK-AP mice ( Fig. 9a ), no such accelerated atrophy of forebrains occurred in male Tau4RΔK-AP mice ( Fig. 9b ). Histological analysis showed similar level of brain atrophy ( Fig. 9c ) and neuronal loss in male Tau4RΔK-AP as compared with that of male Tau4RΔK mice ( Fig. 9d ). No significant changes in accumulation of Aβ plaques ( Fig. 9e ) or activated astrocytes ( Fig. 9g ) were observed in male Tau4RΔK-AP mice. The accumulation of tau aggregates was not significantly altered in male Tau4RΔK-AP mice as compared with that of male Tau4RΔK mice ( Fig. 9f ), indicating that neuritic plaques have little effect on the rate of tau aggregation after its onset. Taken together, these results establish that the neuritic plaque is required for the pathological conversion of wild-type tau. 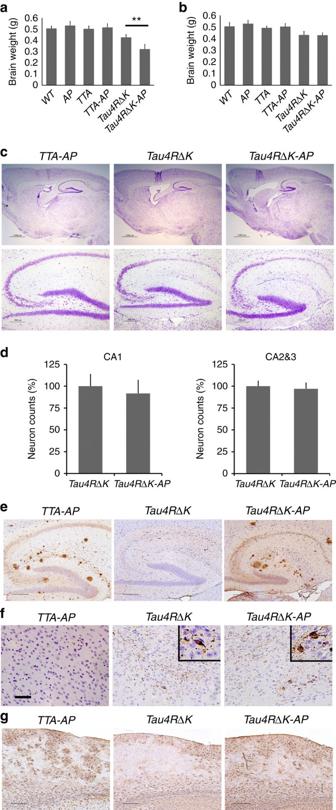Figure 9: Acceleration of onset of tau pathology is dependent on the Neuritic plaque. (a) Brain weight of 12-month-old femalenTG(n=11), AP(n=9), TTA(n=7), TTA-AP(n=7),Tau4RΔK(n=5) andTau4RΔK-AP(n=4) mice. The brain weight ofTau4RΔK-APmice is 25% smaller than that of theTau4RΔKmice at 12 month of age. (one-way analysis of variance, **P=0.002). (b) Brain weight of 12 month-old malenTG(n=11), AP(n=6), TTA(n=6), TTA-AP(n=7),Tau4RΔK(n=5) andTau4RΔK-AP(n=5) mice. No significant difference in brain weight is detected between the maleTau4RΔK-APandTau4RΔKmice at 12 month of age. (c) CV staining of brain sections of 11-month-old maleTTA-AP, Tau4RΔKandTau4RΔK-APmice brains (upper panels; scale bar, 1,000 μm; and hippocampi, lower panels; scale bar, 200 μm). (d) Neuronal cell count of CA1, and CA2&3 region from 11 months old maleTau4RΔK(n=6) andTau4RΔK-AP(n=4) mice. No significant difference was observed between the two mouse lines. (e) Immunostaining of brain sections of 11-month-old maleTTA-AP(n=5), Tau4RΔK(n=5) andTau4RΔK-APmice (n=4) with antibodies (6E10) specific to human Aβ. Scale bars, 200 μm. (f) Immunostaining of brain sections of 11 month-old maleTTA-AP(n=5), Tau4RΔK(n=5), andTau4RΔK-AP(n=4) mice using tau-pS422. Scale bar, 100 μm. (g) Immunostaining of brain sections of 11-month-oldTTA-AP(n=5), Tau4RΔK(n=5) andTau4RΔK-AP(n=4) mice with antibodies specific to GFAP. Scale bars, 200 μm. Figure 9: Acceleration of onset of tau pathology is dependent on the Neuritic plaque. ( a ) Brain weight of 12-month-old female nTG ( n =11) , AP ( n =9) , TTA ( n =7) , TTA-AP ( n =7), Tau4RΔK ( n =5) and Tau4RΔK-AP ( n =4) mice. The brain weight of Tau4RΔK-AP mice is 25% smaller than that of the Tau4RΔK mice at 12 month of age. (one-way analysis of variance, ** P =0.002). ( b ) Brain weight of 12 month-old male nTG ( n =11) , AP ( n =6) , TTA ( n =6) , TTA-AP ( n =7), Tau4RΔK ( n =5) and Tau4RΔK-AP ( n =5) mice. No significant difference in brain weight is detected between the male Tau4RΔK-AP and Tau4RΔK mice at 12 month of age. ( c ) CV staining of brain sections of 11-month-old male TTA-AP, Tau4RΔK and Tau4RΔK-AP mice brains (upper panels; scale bar, 1,000 μm; and hippocampi, lower panels; scale bar, 200 μm). ( d ) Neuronal cell count of CA1, and CA2&3 region from 11 months old male Tau4RΔK ( n =6) and Tau4RΔK-AP ( n =4) mice. No significant difference was observed between the two mouse lines. ( e ) Immunostaining of brain sections of 11-month-old male TTA-AP ( n =5) , Tau4RΔK ( n =5) and Tau4RΔK-AP mice ( n =4) with antibodies (6E10) specific to human Aβ. Scale bars, 200 μm. ( f ) Immunostaining of brain sections of 11 month-old male TTA-AP ( n =5) , Tau4RΔK ( n =5), and Tau4RΔK-AP ( n =4) mice using tau-pS422. Scale bar, 100 μm. ( g ) Immunostaining of brain sections of 11-month-old TTA-AP ( n =5) , Tau4RΔK ( n =5) and Tau4RΔK-AP ( n =4) mice with antibodies specific to GFAP. Scale bars, 200 μm. Full size image Clarification of the key factors contributing to the pathological conversion of wild-type tau, a prion strain or conformation that is perhaps unique to AD [43] , could be instrumental for developing effective therapy for this devastating disease of the elderly. Our findings here establish that the neuritic plaque is required but not sufficient to drive the pathological conversion of wild-type tau. While previous effort primarily employed transgenes expressing tau mutants linked to FTDP-17 (refs 9 , 10 , 11 , 35 , 36 , 37 , 42 ) that are sufficient to aggregate independent of the neuritic plaque, we developed a mouse model expressing human tau repeat domain that is capable of inducing the pathological conversion of mouse wild-type tau only in the presence of the neuritic plaque. Our discovery provides a fundamental paradigm shift and a framework towards identification of risk alleles/factors that play essential roles in the pathological conversion of tau in AD. On the basis of our discovery, we propose here a model ( Fig. 10 ) whereby the β-amyloid dependent formation of neuritic plaque during aging provides the molecular environment to facilitate the biochemical modification of tau within dystrophic neurites. While the neuritic plaque is necessary, it is not sufficient to convert the wild-type tau to a pathological conformation that drives neurodegeneration with ensuing cognitive decline and atrophy of the brain. In addition to the neuritic plaque, we envision a second-risk determinant (here we illustrate with the fragmentation of tau) would be required to drive the pathological conversion of wild-type tau. Thus, we propose that a combination of risk alleles/factors may facilitate the neuritic plaque-dependent pathological conversion of the wild-type tau in LOAD. Genetic studies has identified a series of risk alleles, in addition to ApoE4 allele, that are associated with LOAD [51] , [52] , [53] , [54] . That subsets of individuals whose brains are littered with neuritic plaques remain cognitive normal [22] , [23] , [24] can be explained by our ‘two-hit’ hypothesis because they fail to harbour another risk allele that is required to drive the conversion of tau. Moreover, our model is also consistent with the long pre-symptomatic phase seen in LOAD [55] , [56] during which time neuritic plaques accumulate because until the second-risk determinant is activated, tau remains unconverted. Likewise, our model predicts that cognitive decline in LOAD would be correlated with tau pathology rather than with neuritic plaques because once initiated, the tau aggregates are sufficient to propagate and spread throughout the brain via neuronal circuits and drive neuronal loss with ensuing cognitive decline. Thus, we believe that the pathogenesis of LOAD is a multifactorial problem initiated by the age-dependent formation of the neuritic plaque and activation of a variety of potential risk determinants to drive the pathological conversion of tau ( Fig. 10 ). 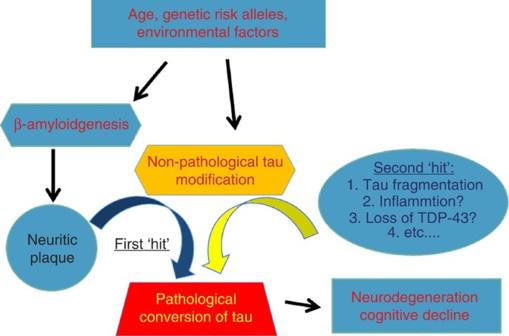Figure 10: A multifactorial Model for LOAD. Diagram depicting that the neuritic plaque is required, but insufficient for the pathological conversion of tau. A second ‘hit’ involving a variety of risk alleles/factors, would be necessary to facilitate the neuritic plaque-dependent pathological conversion of the wild-type tau in LOAD. Figure 10: A multifactorial Model for LOAD. Diagram depicting that the neuritic plaque is required, but insufficient for the pathological conversion of tau. A second ‘hit’ involving a variety of risk alleles/factors, would be necessary to facilitate the neuritic plaque-dependent pathological conversion of the wild-type tau in LOAD. Full size image From a therapeutic perspective, our model first predicts that therapies designed to prevent the conversion of tau would be most beneficial because the presence of neuritic plaques, in the absence of tau aggregates will not be sufficient to drive neuron loss. Our novel mouse model exhibiting age- and neuritic plaque-dependent tau pathology will now provide an invaluable platform for testing a variety of risk alleles/factors that may be relevant for the pathological conversion of tau. While a three-dimensional human neural cell culture system displaying Aβ and tau pathologies [57] is a very useful tool for in vitro drug screening, our model exhibiting age-dependent development of neuritic plaques and tau pathologies that drives the progressive loss of neuron will be an essential in vivo tool for drug discovery programs designed to attenuate neurodegeneration for LOAD. Second, our model predicts that anti-amyloid therapies directed at early pre-symptomatic AD long before the pathological conversion of tau would slow disease by delaying the onset of tau pathology. In retrospect, perhaps it was not too surprising that outcomes of clinical trials with anti-amyloid agents in humans have been disappointing [58] , [59] , [60] , [61] when delivered during a time when the conversion of tau has already initiated. Finally, our model predicts that a combinatorial therapy designed to prevent both neuritic plaque formation as well as pathological conversion of tau may provide optimal benefit for LOAD. Generation of transgenic mice To generate tau transgenic mice, DNA fragments encoding wild-type and ΔK280 mutant four-repeat domains of tau (TauRD, that is,Q244-E372) were subcloned into a previously characterized moPrP-tetP vector [48] , which expresses the gene consistently in neurons under the control of tTA proteins. The DNA was microinjected into C57BL/6 X SJL F2 mouse embryos (University of Michigan transgenic facility) to produce transgenic mice carrying wild-type ( TetO-TauRD) or mutant ( TetO-TauRDΔK ) Tau fragment with regulatory element, moPrP-tetP promoter. Subsequently, these mice were crossbred with CamKII-tTA mice to bring the Tau transgene under the control of tet-off CamKII promoter [62] ( Tau4R and Tau4RΔK mice). Doxycycline hydrochloride, dissolved in water to final concentration of 20 mg ml −1 and sterilized by filtration with 0.22 μm filter, was supplied in the drinking water to suppress the exogenous Tau expression during early development. During gestation and before weaning, the mice were raised in the presence of 50 μg ml −1 doxycycline hydrochloride. We crossbred CamKII-tTA;TetO-TauRD or CamKII-tTA;TetO-TauRDΔK mice with APP swe ;PS1ΔE9 mice [49] to generate APP swe ;PS1ΔE9;CamKII-tTA;TetO-TauRD (Tau4R-AP ) and APP swe ;PS1ΔE9;CamKII-tTA;TetO-TauRDΔK (Tau4RΔK-AP) mice that develop both Tau pathology and Aβ amyloidosis; Tau4R or Tau4RΔK, CamKII-tTA (TTA), APP swe ;PS1ΔE9;CamKII-tTA (TTA-AP), APP swe ;PS1ΔE9 (AP) and non-transgenic littermates were used as controls. The brains of mice at various ages were collected, weighed and processed for biochemical, histological and immunohistochemical analysis. All mice were maintained under 12L:12D cycle in centralized animal housing facility programme managed by Research Animal Resources (RAR) at the Johns Hopkins University. All animal procedures were in strict accordance with the National Institutes of Health Guide for the Care and Use of Laboratory Animals and were approved by the Johns Hopkins University Animal Care and Use Committee. Immunoblots and antibodies Immediately after killing, mouse brains were dissected [63] in the specific brain regions olfactory bulb, hippocampus, striatum, cortex, midbrain, brain stem, cerebellum and the rest. Proteins of each region were extracted with RIPA buffer (10 mM Tris-Cl (pH 8.0), 1 mM EDTA, 0.5 mM EGTA, 1% Triton X-100, 0.1% sodium deoxycholate, 0.1% SDS and 140 mM NaCl) containing 1 × complete protease inhibitor cocktail (Roche, Indianapolis, IN). The protein concentrations in the supernatants were determined by the BCA method (Pierce Chemical Co., Rockford, IL) and equal amounts of protein lysates ( ∼ 20 μg per lane) resolved on 4–12% Bis-Tris SDS–PAGE gels with MES running buffer, then transferred to polyvinylidene difluoride (Invitrogen, Carlsbad, CA) membranes, and probed with following antibodies: anti-human tau polyclonal antiserum KJ9A (1:5,000; A0024, Dako Cooperation, Carpinteria, CA); Purified anti-Tau 316–355 monoclonal antibody 77G7 (1:1,000; BioLegend, San Diego, CA); rabbit anti-APP C-terminal (1:2,000; AB5352, Chemicon); monoclonal antibody against synaptophysin (1:1,000; AB8049, Abcam, Cambridge, MA); rabbit anti-GAPDH antiserum (1:5,000; G9545, Sigma); and monoclonal anti-β-tubulin III antiserum (1:10,000; T2200, Sigma). Immunoblots were developed using enhanced chemiluminescence method (Millipore Corp., MA). Histology and immunohistochemical analysis For the histological and immunohistochemical analysis mice were anaesthetised and killed by decapitation at different ages [64] ; brains were removed and weighed. Hemibrains were fixed by submerging into 4% paraformaldehyde (PFA) in PBS, embedded into the paraffin, sectioned in sagittal plane and processed. For histological analyses, 10 μm brain sections were stained with hematoxylin and eosin or Cresyl violet. Hirano silver stain utilized Hirano’s modification of the Bielschowsky method [65] , [66] . Briefly, 200 ml of ammonium hydroxide were evaporated under vacuum for 30 min. Sections were deparaffinized for 10 min and placed in 20% sliver solution for 30 min. After a rinse in dH 2 O, slides were transferred to ammoniacal solution (200 ml 20% silver nitrate solution with drops of evaporated ammonium hydroxide) for 15 min. Slides were washed in dH 2 O with four drops of ammonium hydroxide, transferred to ammoniacal solutions with three drops of developer, rinsed in dH 2 O and fixed in 1% sodium thiosulfate for 1 min. Finally the slides were washed with dH 2 O, dehydrated, cleared and mounted. Gallyas silver staining was modified from Braak [67] and performed as follows. Slides were deparaffinized and dipped in 5% periodic acid. After a brief wash with water, the slides were incubated for 1 min in silver iodide solution (290 ml dH 2 O, 12 g sodium hydroxide, 30 g potassium iodide, 10 ml 1%silver nitrate). After a wash in 0.5% acetic acid (2 × 5 min), slides were rinsed with dH 2 O and developed for 10–20 min in physical developer solution. After a 5 min wash in 0.5% acetic acid and dH 2 O, slides were incubated in 0.1% gold chloride for 5 min. Next, the slides were rinsed in dH 2 O and fixed in 1% sodium thiosulfate for 5 min. For counterstaining, the slides were dipped in 0.1% nuclear fast red for 2 min before getting washed in tap water, dehydrated and mounted. The Congo Red stain was performed as followed. Slides were deparaffinized, stained in congo red solution (50 ml 80% alcohol, 0.15 g Congo red, 0.15 g sodium chloride, 0.5 ml 1% sodium hydroxide) for 10 min and rinsed in dH 2 O. The stain was differentiated by dipping the slides 5–10 times in alkaline alcohol solution (100 ml 50% alcohol, 1 ml 1% sodium hydroxide), rinsed in water, dehydrated and mounted. For the Thioflavin-T staining slides were deparaffinized and hydrated. Slides were incubated in 0.25% potassium permanganate solution for 5 min, transferred to 1% potassium-diulfate and oxcalic acid for 5 min and incubated in 0.02% Thioflavin-T for 8 min. Slides were dehydrated and mounted with aqueous mounting medium for fluorescence. The area size of hippocampus, cortex and cerebellum in sagittal sections at 2 mm from the midline of the brains were measured by the ImageJ program. Semiquntitative score of Tau tangles was evaluated in low power ( × 200) microscope field as described previously [68] . Score was indicated as: 0, no tangle; 1, 1–5 tangles per field; 2, 6–15 tangles per field; and 3, >15 tangles per field. For immunohistochemical analysis, antigen retrieval was performed with 10 mM citrate buffer (pH 6.0) for an efficient epitope exposure to the antibodies; endogenous peroxidase was quenched by treating the paraffin sections with 0.3% H 2 O 2 ; and nonspecific binding of antibodies was eliminated using blocking buffer (10% normal goat serum in PBS with 0.3% Triton-X) for 1 h at room temperature. The primary antibody prepared in blocking buffer was applied for overnight at 4 o C, followed by a secondary antibody for 30 min incubation at room temperature. For the secondary antibody and avidin-biotinylated peroxidase system, we used the Vectastain Universal Elite ABC kit (Vector Laboratories). Brain sections were stained with: antiserum against Aβ peptides 6E10 (1:1,000; SIG-39300, Covance); antiserum against pan-tau antibody K9JA (1:1,000; A0024, Dako Cooperation, Carpinteria, CA); mouse monoclonal antiserum against phosphorylated tau CP13 (1:1,000; Tau pS202) and PHF-1 (1:1,000, Tau pS396/S404) (gifts of P. Davis, Albert Einstein College of Medicine); rabbit antiserum against phosphorylated T231(1:1,000; 44746G, Invitrogen, Carlsbad, CA), phosphorylated S262 (1:1,000; 44705G, Invitrogen, Carlsbad, CA) phosphorylated S396 (1:1,000; 44752, Invitrogen, Carlsbad, CA) and S422 of tau (1:2,000; 44764G, Invitrogen, Carlsbad, CA); ubiquitin, Microtubule-associated protein 2 (Map2, 1:1,000; AB5622, Millipore), phosphorylated neurofilament (Smi31, 1:1,000; BioLegend, San Diego, CA), neurofilaments in axons (Smi312, 1:1,000; BioLegend, San Diego, CA), Neurofilament triplet H protein (NF-H; 1:1,000, Sigma, Saint Louis, MO, USA), polyclonal antiserum against GFAP (Z0334, Dako Cooperation, Carpinteria, CA); polyclonal antiserum against microglial (IBA1, CP290, Biocare Medical, CA), and monoclonal antibody against NeuN (MAB377, Millipore). Sections for immunofluorescence were examined under a Zeiss LSM 510 laser scanning fluorescence confocal microscope. Z-stack projections were made from serial scanning every 1 μm to reconstruct the Aβ plaques. Data analysis All data were analysed statistically by unpaired Student’s two-tailed t -test or one-way analysis of variance with Tukey’s correction for multiple comparisons using GraphPad Prism version 6.0 f for Mac, GraphPad Software, La Jolla, CA, USA. In all tests, values of P <0.05 were considered to indicate significance. Data availability The authors declare that all data supporting the findings of this study are available within the article and its Supplementary Information files or from the authors on request. How to cite this article: Li, T. et al . The neuritic plaque facilitates pathological conversion of tau in an Alzheimer’s disease mouse model. Nat. Commun. 7:12082 doi: 10.1038/ncomms12082 (2016).